Eutrophication will increase methane emissions from lakes and impoundments during the 21st century Lakes and impoundments are an important source of methane (CH 4 ), a potent greenhouse gas, to the atmosphere. A recent analysis shows aquatic productivity (i.e., eutrophication) is an important driver of CH 4 emissions from lentic waters. Considering that aquatic productivity will increase over the next century due to climate change and a growing human population, a concomitant increase in aquatic CH 4 emissions may occur. We simulate the eutrophication of lentic waters under scenarios of future nutrient loading to inland waters and show that enhanced eutrophication of lakes and impoundments will substantially increase CH 4 emissions from these systems (+30–90%) over the next century. This increased CH 4 emission has an atmospheric impact of 1.7–2.6 Pg C-CO 2 -eq y −1 , which is equivalent to 18–33% of annual CO 2 emissions from burning fossil fuels. Thus, it is not only important to limit eutrophication to preserve fragile water supplies, but also to avoid acceleration of climate change. The importance of lakes and rivers in the global carbon cycle is well established [1] , [2] , [3] . Local, regional, and global emission estimates of the carbonic greenhouse gases (GHGs), methane (CH 4 ) and carbon dioxide (CO 2 ), are reported regularly [1] , [2] , [4] , [5] with estimates of nitrous oxide (N 2 O), another potent GHG produced in aquatic systems, also occasionally reported [6] . One of the most recent estimates of global GHG emissions from lakes and impoundments [7] found that while absolute emission of CO 2 is 5–10 times more than that of CH 4 and N 2 O (in Tg of carbon (C) or nitrogen (N) per year), about 72% of the climatic impact of GHG emissions (in CO 2 -equivalents) from lakes and impounded waters is due to CH 4 . This is because CH 4 is up to 34-times more potent as a GHG than CO 2 and is responsible for approximately 20% of the overall additional atmospheric radiative forcing observed since 1750 [8] . This recent finding regarding the importance of aquatic CH 4 emissions [7] contradicts earlier reports that CH 4 and CO 2 contributed equally to the global warming potential of GHG emissions from lakes and impoundments [2] , [4] , [6] . These previous estimates, however, were based on a simplistic upscaling method of extrapolating average observed emission rates to global lake and impoundment surface area without regard for driving mechanisms. The use of this type of upscaling, rather than a process-based approach, may be the cause for the large uncertainties surrounding global aquatic CH 4 emissions [9] . While CH 4 emission rates are known to be controlled by a wide range of factors including lake depth [10] and sedimentation rates [11] , to name a few, incorporation of drivers into approaches for estimating CH 4 emissions has been limited by the lack of world-wide data on these factors. Remote sensing approaches are beginning to fill data gaps, however, and global datasets are now available for lake size and productivity, two important drivers of CH 4 emissions [12] . DelSontro et al. [7] used these global datasets, along with >8000 GHG flux measurements, and modeled emission rates as a function of system productivity and lake size. They found, as did a smaller study of impoundments [13] , that not only was CH 4 the most important GHG emitted from aquatic systems in terms of climate impact, but that it rises exponentially with lake and impoundment chlorophyll a (chla) concentration, a proxy for productivity [7] . This is consistent with multiple lake studies showing that CH 4 emissions positively correlate with productivity variables such as total phosphorus (TP) and chla [5] , [10] , [13] , [14] , [15] , [16] . Ultimately, these relationships reflect the link between an increase in organic substrate and enhanced rates of methanogenesis in productive aquatic systems [14] , [17] , [18] . This is an important finding because the productivity of inland waters is projected to increase in the coming decades. 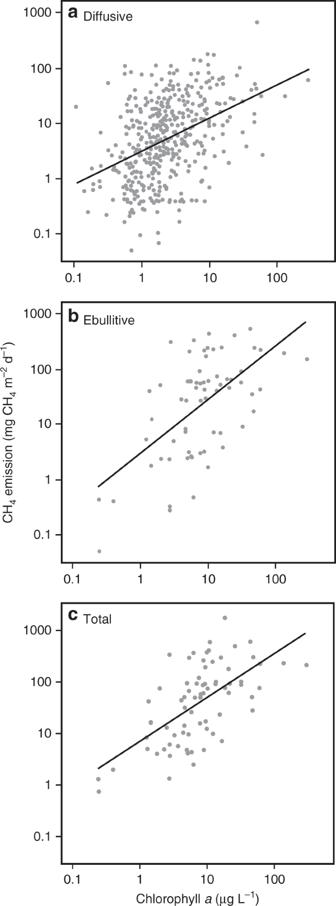Fig. 1 Relationships between CH4flux rates and productivity measured as the concentration of chlorophylla(chla) in the water column of lakes and impoundments. Solid lines are regression relationships.aDiffusive flux is the flux rate from the water to the atmosphere driven by super-saturation in the water column.bEbullitive flux is that emitted by the formation of bubbles transported to the surface.cTotal flux is the sum of both diffusive and ebullitive flux. Note: panelashows only the relationship between diffusive CH4flux and chla concentration, whereas the predictive model for diffusive flux includes both a lake size and chla effect (Table3) Three distinct mechanisms are expected to induce increases in aquatic productivity over the next century (Table 1 , Supplementary Table 1 ). First, increased human populations (+37% by 2050, +50% by 2100 [19] ) will augment the release of sewage and agricultural fertilizers to inland waters by an estimated 1.23×–1.97× (e.g., increase by up to a factor of 1.97, expressed as 1.97× hereafter) by 2050 and 1.41×–3.19× by 2100 [20] , [21] , [22] . On a global scale, the spatial distribution of agricultural nutrient use correlates with that of surface water [23] , presumably because sustained crop growth requires both nutrients and ample water; therefore, increased global nutrient use is likely to affect inland surface waters. Second, increased storms and runoff will enhance nutrient losses from land by a mean 1.14× over the same period [24] , [25] , further increasing nutrient delivery to inland waters. Third, warming surface waters will increase global aquatic primary production by ~1.30× by 2100 [26] . These increases in eutrophication and consequent CH 4 production will be augmented by the 1.10× net global expansion in lakes and impoundment spatial extent [2] , [26] , [27] expected over the 21st century, resulting in more CH 4 -emitting surface waters. A further increase we cannot assess is enhanced nutrient concentrations in warm regions resulting from increased evaporation, which may be regionally important [26] , [28] , but has not been estimated globally. Projected increases in lake eutrophication are supported by a recent report that the fraction of lakes in the US that are oligotrophic decreased  from 25% of all surveyed lakes to 7% over just a 5-year period (2007–2012) [29] . Depending on the trajectory of human population growth and changes in climate and weather, multiplying nutrient effects by exacerbating factors (Table 1 , Supplementary Table 1 ) shows that productivity of lakes and impoundments will likely increase 1.37×–3.10× by 2050 and 2.17×–4.91× by 2100. Table 1 Changes driving expanded eutrophication and rising CH 4 emissions from lakes and impoundments during the 21st century Full size table Here, we use the relationship between CH 4 emission rates and chla reported in DelSontro et al. [7] (Fig. 1 ) to predict the effect of increased eutrophication of the earth’s lakes and impoundments on CH 4 emissions. We simulated four levels of increased TP concentration (1.5× , 2× , 2.5× , and 3× that of current levels) that are conservatively within the magnitude of increase predicted by diverse authors and models through 2100 (Table 1 ). We further simulated a future where improved nutrient management results in TP concentrations 0.75× that of current levels. We calculated the corresponding changes in chla (0.8× , 1.3× , 1.7× , 2.0× , and 2.2× that of current levels) using a non-linear TP—chla relationship derived from published data [30] (Supplementary Figure 1 ). These relationships were applied to the global lake and impoundment surface area reported in Downing et al. [31] . The current global distribution of chla in lakes and impoundments was estimated using satellite-based measurements of chla in 80,000 lakes around the world [32] . Our simulation results indicate that enhanced eutrophication will increase CH 4 emissions from lakes and impoundments by 30–90% over the next century. Fig. 1 Relationships between CH 4 flux rates and productivity measured as the concentration of chlorophyll a (chla) in the water column of lakes and impoundments. Solid lines are regression relationships. a Diffusive flux is the flux rate from the water to the atmosphere driven by super-saturation in the water column. b Ebullitive flux is that emitted by the formation of bubbles transported to the surface. c Total flux is the sum of both diffusive and ebullitive flux. Note: panel a shows only the relationship between diffusive CH 4 flux and chla concentration, whereas the predictive model for diffusive flux includes both a lake size and chla effect (Table 3 ) Full size image Enhanced CH 4 emissions due to future productivity increases Our model indicates that future eutrophication of the world’s lakes and impoundments will increase diffusive, ebullitive, and total CH 4 emissions (Fig. 2 ). Assuming a 3× increase in TP concentrations, diffusive emissions may increase from current levels (28 Tg C-CH 4 y −1 ) up to 45 Tg CH 4 -C y −1 , representing a 60% increase in emissions. 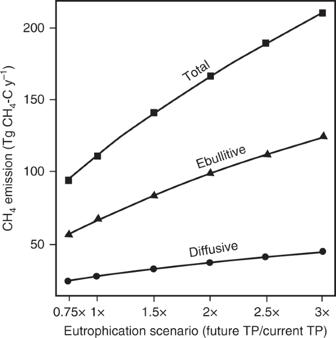Fig. 2 Simulated future global emissions of CH4calculated at multiple levels of increased eutrophication driven by accelerated TP loading to lakes and impoundments (see Methods). The scenarios are based on a review of the published literature and reflect future TP concentrations that are 0.75, 1.5, 2, 2.5, and 3× greater (i.e., 0.75×, 1.5×, 2×, 2.5×, 3×) than current levels (1×), as indicated onx-axis. Simulated TP concentration was converted to chlorophylla(chla) using published data (see Methods and Supplementary Figure 1) resulting in future chla concentrations that are 0.8, 1.3, 1.7, 2.0, and 2.2× that of current levels. CH4emissions were predicted from lake surface area and/or chla Ebullition and total (diffusive + ebullitive) CH 4 emission rates are more sensitive to enhanced eutrophication and will nearly double (mean increase of 1.86×) in a future environment with 3× greater nutrient loading to lakes and impoundments (Supplementary Table 2 ). Fig. 2 Simulated future global emissions of CH 4 calculated at multiple levels of increased eutrophication driven by accelerated TP loading to lakes and impoundments (see Methods). The scenarios are based on a review of the published literature and reflect future TP concentrations that are 0.75, 1.5, 2, 2.5, and 3× greater (i.e., 0.75×, 1.5×, 2×, 2.5×, 3×) than current levels (1×), as indicated on x -axis. Simulated TP concentration was converted to chlorophyll a (chla) using published data (see Methods and Supplementary Figure 1) resulting in future chla concentrations that are 0.8, 1.3, 1.7, 2.0, and 2.2× that of current levels. CH 4 emissions were predicted from lake surface area and/or chla Full size image At current productivity levels, we find that total CH 4 emissions (112 Tg C-CH 4 y −1 ) are approximately 25% higher than the latest global estimates for lakes and impoundments (88.7 Tg C-CH 4 y −1 ) [9] , which was based on a synthesis of measurements from mostly northern systems (>50°N) that used the traditional upscaling approach. Under a scenario of a tripling of nutrient loading, we could find the aggregate of global lakes and impoundments emitting more than double the current global estimate. More concerning yet is that even at the smallest increase in TP suggested by the literature (1.5×) we would see total global lake CH 4 emissions rise to 141 Tg C-CH 4 y −1 , equivalent to global emissions from wetlands, which is the current single largest source of atmospheric CH 4 (139 Tg C-CH 4 y −1 ) [9] . A tripling of nutrient loading could result in total lake CH 4 emissions being 1.5× higher than the current wetland emission estimate. It is possible, though unlikely, that improved nutrient management practices could reverse the eutrophication of lakes and impoundments, thereby reducing CH 4 emissions. For example, a 25% reduction in global TP loading (0.75×) could prevent the emissions of 17 Tg CH 4 -C y −1 (Fig. 2 , Supplementary Table 2 ). While a net reduction in nutrient loading is unlikely to occur on a global scale due to increasing population, it may be realized regionally or for individual water bodies and could be included in the cost/benefit analysis of nutrient management programs [33] . Our literature review indicates that global TP loading of inland waters will increase over the 21st century, stimulating aquatic productivity and CH 4 emissions. We find that these changes could result in total lake CH 4 emissions having an atmospheric impact equivalent to 18–33% of that from current fossil fuel CO 2 emissions (Table 2 ). In fact, the net increase in CH 4 emissions due to projected nutrient loading alone would have an atmospheric effect more than increased CO 2 emissions from land use change (i.e., conversion of forests to agriculture) or up to half of the global oceanic and land carbon sinks (Table 2 [3] , [34] ). The projected CH 4 emission increases reported here  should be considered minimal because they do not account for the synergistic interaction between nutrients and water temperature on CH 4 production rates [39] , future increases in impounded area [27] , or the effect of eutrophication on CH 4 emissions from streams, rivers, small ponds, and wetlands. Eutrophication is considered to be one of the world’s most pressing environmental issues [35] and, if it continues, will exacerbate global climate change. Table 2 Projected increases in CH 4 emissions from lakes and impoundments as compared to major global CO 2 sources and sinks Full size table Experimental design We simulated future TP loadings to lakes and impoundments that are 0.75×, 1.5×, 2×, 2.5×, or 3× that of current loading, a conservative set of scenarios relative to our literature review which indicated that TP may increase nearly 5× relative to current levels by 2100 (Table 1 , Supplementary Table 1 [20] , [22] , [24] ,] [36] ). Changes in TP concentration were translated to changes in chlorophyll a (chla) concentration using the non-linear TP—chla relationship derived from the data in McCauley et al. [30] (Supplementary Figure 1 ) and an estimate of the current global chla distribution in lakes and impoundments. The global distribution of chla in lakes and impoundments was derived from satellite-based chla measurements of 80,000 lakes around the world [32] . We combined these data with an estimate of the size distribution of lakes and impoundments [31] to generate a joint lake-size by productivity distribution for the worlds lakes and impoundments. Although several global lake-size distributions are available in the literature, all of them offer very similar conclusions. The data were aggregated into twenty 5 μg L −1 chla bins and nine lake-size bins ranging from 0.001 to >100,000 km 2 . These TP loading scenarios (0.75×, 1.5×, 2×, 2.5×, or 3×) resulted in future chla concentrations that are, on average, 0.8×, 1.3×, 1.7×, 2.0×, and 2.2× that of the current global chla distribution. We propagated each of these chla distributions across the joint lake-size by chla distribution, resulting in five new distributions reflecting differing levels of eutrophication (Supplementary Data 1 ). We calculated global CH 4 emissions for each scenario using statistical models relating diffusive, ebullitive, and total CH 4 emission rates to lake size and/or water column chla content (Table 3 ). First, we calculated the mean areal emission rate (mg CH 4 -C m −2 d −1 ) for each lake-size by chla bin. Next, we multiplied the predicted areal emission rate for each bin by the total water body surface area corresponding to the bin. Finally, we summed the emissions across bins and scaled the result to an annual emission estimate for each emission mechanism (i.e., diffusive, ebullitive, and total emissions). Table 3 Statistical models used to predict methane (CH 4 ) emission rates Full size table The range of TP and chla concentrations in the most extreme 3× simulation (11–1669 µP L −1 and 5.7–216 µg L −1 , respectively) were well within the range of values included in the literature used to parameterize the statistical models [7] (Fig. 1 ). Statistical uncertainty in the model predictions was propagated through the calculations and is presented as 95% confidence intervals in Supplementary Table 2 and Supplementary Data 1 . The statistical models used to predict CH 4 emission rates do not include an effect for water body origin (i.e., natural vs constructed) because of insufficient data coverage across the range of covariates for both system types. There is little evidence in the literature that suggests CH 4 emission rates differ between natural lakes and impoundments, after system size and productivity are accounted for. Furthermore, impoundments constitute a small fraction of total inland water surface area [31] , therefore any systematic difference in the response of CH 4 emission rate to size or productivity between natural lakes and impoundments will likely have little effect on cumulative global CH 4 emissions from lentic waters. Statistical analysis The models used to upscale lake and impoundment methane (CH 4 ) emissions are presented in DelSontro et al. [7] and are reproduced in Table 3 . The models predict CH 4 emission rates (mg CH 4 -C m −2 d −1 ) from lake size (km 2 ) and/or chla (µg L −1 ).